Ranking in interconnected multilayer networks reveals versatile nodes The determination of the most central agents in complex networks is important because they are responsible for a faster propagation of information, epidemics, failures and congestion, among others. A challenging problem is to identify them in networked systems characterized by different types of interactions, forming interconnected multilayer networks. Here we describe a mathematical framework that allows us to calculate centrality in such networks and rank nodes accordingly, finding the ones that play the most central roles in the cohesion of the whole structure, bridging together different types of relations. These nodes are the most versatile in the multilayer network. We investigate empirical interconnected multilayer networks and show that the approaches based on aggregating—or neglecting—the multilayer structure lead to a wrong identification of the most versatile nodes, overestimating the importance of more marginal agents and demonstrating the power of versatility in predicting their role in diffusive and congestion processes. A comprehensive definition of centrality has driven the interest of sociologists for several decades [1] , [2] , [3] , although, intriguingly, the result is not unique. Many different measures, depending on the application of interest, have defined centrality in terms of activity, control, communicability or independence [4] . Centrality measures are useful to identify proteins crucial for the survival of the cell [5] , design optimal network topologies for local search with congestion [6] , design efficient ways in which to engineer the structure of the network [7] , identify influential spreaders [8] , drive the network towards a desired state [9] , or mitigate the cascading failures of technological networks [10] and identify potential drug targets in a signalling network of human cancer [11] . Although probably, the most famous, by use, measure of centrality is PageRank [12] , the ranking measure operating behind the universal search engine of Google. It has been a common practice, in network theory, to assume that nodes are linked by a single type of static edge that encapsulates their interactions, although in a myriad of scenarios this assumption oversimplifies the complexity of the network. Accounting for different types of interactions between nodes can be nowadays correctly analysed in the framework of multilayer networks [13] , [14] , [15] , [16] , [17] . A schematic of an interconnected multilayer network is shown in Fig. 1 (see Supplementary Note 1 for additional real-world examples and Supplementary Fig. 1 for additional synthetic examples). Neglecting the existence of multiple relationships between nodes, or aggregating such relationships to a single weighted network, alters the topological and dynamical properties of the full system [15] , [18] , [19] , [20] and the importance of the nodes with respect to the whole structure [21] , [22] , [23] , [24] , [25] . 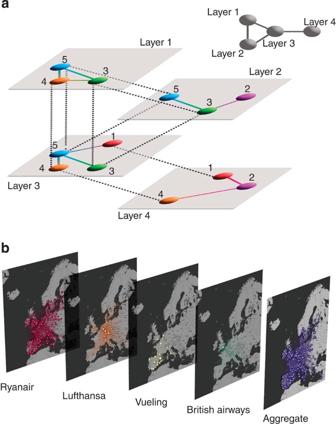Figure 1: Multilayer networks. (a) Representation of a multilayer network with five nodes in four layers. Each layer represents a different level of interaction or relationship between nodes. Nodes might (or might not) exist in all layers. The coupling between layers (dotted lines) determines the network of networks (see the top-right inset) and interlayer links might exist between nodes and their counterparts in other layers (as in multiplex-like networks) or between different nodes in different layers (as in general multilayer networks). Such information is fully encoded in a rank-4 adjacency tensor. (b) Multilayered visualization of an empirical interconnected multiplex network, where interlayer connections are present but not shown for simplicity. Layers correspond to flight routes operated by different air companies between European airports26. Map tiles By Stamen Design, under CC BY 3.0. Data by OpenStreetMap, under CC BY SA. Figure 1: Multilayer networks. ( a ) Representation of a multilayer network with five nodes in four layers. Each layer represents a different level of interaction or relationship between nodes. Nodes might (or might not) exist in all layers. The coupling between layers (dotted lines) determines the network of networks (see the top-right inset) and interlayer links might exist between nodes and their counterparts in other layers (as in multiplex-like networks) or between different nodes in different layers (as in general multilayer networks). Such information is fully encoded in a rank-4 adjacency tensor . ( b ) Multilayered visualization of an empirical interconnected multiplex network, where interlayer connections are present but not shown for simplicity. Layers correspond to flight routes operated by different air companies between European airports [26] . Map tiles By Stamen Design, under CC BY 3.0. Data by OpenStreetMap, under CC BY SA. Full size image Despite of their ubiquity, multilayer networks are still poorly understood. Here we exploited a recent mathematical grounded formalism that uses a tensorial representation of multilayer networks to determine their most central nodes with respect to specific established definitions. In the case of multilayer networks, the corresponding representation is a rank-4 tensor encoding a directed, weighted, connection between node i from layer α to any other node j in any other layer β (see Supplementary Note 2 for details about notation and on the tensorial nature of adjacency tensors). Although it is difficult to represent such a four-dimensional object, it can be thought as composed by two-dimensional slices along the third dimension, representing intralayer connections between nodes within the same layer α , together with two-dimensional slices along the fourth dimension, representing interlayer connections between nodes laying on different layers. This topology and the dynamics of processes on top of it make multilayer networks unique entities with new structural and dynamical properties to be unveiled. It is worth remarking that the monoplex adjacency tensor can be interpreted as a linear transformation which, given a vector (or 1—form) representing a node, returns another vector (or 1—form) with the set of their adjacent nodes. Thus, the only acceptable representation for the monoplex adjacency object is a 1—covariant and 1—contravariant tensor. Likewise, the multilayer adjacency tensor transforms a node in one layer into the set of adjacent nodes, keeping also the information of which layer they belong to, thus a 2—covariant and 2—contravariant tensor is needed. Our results show that calculating the centrality of nodes in each network of the multilayer structure separately or aggregating the information to a single network inevitably leads to misleading results. The tensorial formulation of multilayer networks allows to overcome such limitations and to generalize widely adopted centrality measures (see Supplementary Note 3 ) capturing the importance of nodes in real interconnected topologies, such as social, transportation and biological networks. We demonstrated that our framework provides new insights in empirical networks, which are inherently multilayer, and that accounting for the interconnected structure is an essential requirement to identify key actors (versatile nodes) in systems exhibiting complex relationships. Moreover, versatility is a good predictor for diffusive and congestion processes in multilayer networks. Eigenvector versatility Focusing on ranking the nodes of the multilayer network according to their central role, we have revisited several definitions and adapted them to the new framework. One of the widest adopted measures of centrality in networks is based on an iterative procedure assigning to each node a score that is the sum of the scores of its neighbours. Mathematically, this is equivalent to calculate the largest eigenvalue and the corresponding eigenvector of the adjacency matrix. In the case of interconnected networks, a formally similar procedure is introduced (see Supplementary Note 4 ) to calculate the leading eigentensor Θ iα of as the solution of the tensorial equation [14] where λ 1 is the largest eigenvalue. Here, Θ iα encodes the eigenvector versatility of each node ( i ) in each layer ( α ) when accounting for the whole interconnected structure. The versatility of each node is obtained by aggregating over layers the centrality of each node in each layer computed using the full multilayer structure, by θ i =Θ iα u α , where u α is the rank-1 tensor with all components equal to 1. The choice of this aggregation corresponds to a maximum entropy principle, a reasonable choice when no specific criteria about the importance of layers is considered. When other information is considered, and used to weight layers, it is possible to obtain specific weighted aggregations as discussed in Solá et al . [22] . PageRank versatility Google’s PageRank centrality [12] is a variant of the previous definition, and corresponds to the steady-state solution of the master equation of a random walk where the walker jumps to a neighbour with rate r and teleport to any other node in the network with another rate r ′. We also extended this concept to PageRank versatility of interconnected multilayer networks, where the teleportation might occur to any other node in any layer, and we directly validated our theoretical predictions against simulations (see Supplementary Note 3 for details). Similarly, other measures such as hub/authority, Katz and shortest-path-based (betweenness) versatilities have been described using the tensorial formalism presented above (see full description in Supplementary Note 3 ). It is worth noting that, in general, the calculation of centrality in each layer separately and its subsequent aggregation may lead to misleading results, because the nonlinear competition between layers is difficult to be accounted for a posteriori . A representative example is shown in Fig. 2 (see Supplementary Fig. 1 and Supplementary Note 5 for additional examples). 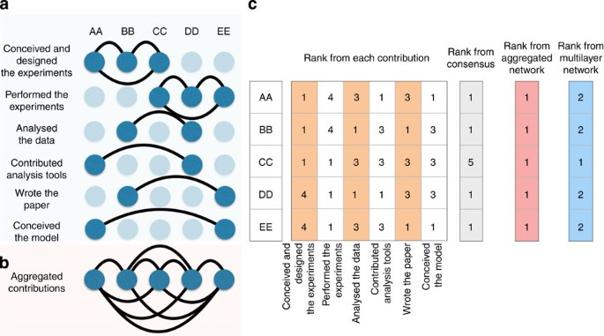Figure 2: Versatility compared with centrality. Here we designed an example of authors’ contributions to a research article. In particular, we consider five authors (AA, BB, CC, DD and EE) and their corresponding contributions. Each contribution represents one layer of a multilayer network (shown ina), where nodes are the above authors. In each layer, a clique is built with all authors participating in the corresponding activity, because we do not have more information about its specific interactions within this contribution category. We show in (b) the network resulting by aggregating the multilayer information: in this case, all authors are linked with each other with the same weight. We show in (c) a table where columns report the rank of each author in each layer separately, obtained using eigenvector centrality: given the multivariate information, we employ a consensus to establish the overall ranking. The result could depend on the choice of the heuristic; however, most of them will assign to all authors the same score. Interestingly, versatility and a weighted (per link) consensus (seeSupplementary Note 5), will rank author CC first. Therefore, four authors out of five are central in this network and it is not possible to remove this ambiguity by calculating centrality in the aggregated network: in fact, all nodes in a clique have the same centrality and all have rank 1. Conversely, the multilayer analysis provides a unique versatile (most central) author, CC, solving the ambiguity raising with classical approaches. CC contributed only in two layers, at variance with the other authors who contributed in three layers, and therefore she is under-represented and consequently under-ranked when heuristics descriptors are employed. However, after a more careful inspection, CC is the only author bridging the two layers with the largest number of contributions and for this reason her role must be more central than other authors, even if they contributed in more layers. Figure 2: Versatility compared with centrality. Here we designed an example of authors’ contributions to a research article. In particular, we consider five authors (AA, BB, CC, DD and EE) and their corresponding contributions. Each contribution represents one layer of a multilayer network (shown in a ), where nodes are the above authors. In each layer, a clique is built with all authors participating in the corresponding activity, because we do not have more information about its specific interactions within this contribution category. We show in ( b ) the network resulting by aggregating the multilayer information: in this case, all authors are linked with each other with the same weight. We show in ( c ) a table where columns report the rank of each author in each layer separately, obtained using eigenvector centrality: given the multivariate information, we employ a consensus to establish the overall ranking. The result could depend on the choice of the heuristic; however, most of them will assign to all authors the same score. Interestingly, versatility and a weighted (per link) consensus (see Supplementary Note 5 ), will rank author CC first. Therefore, four authors out of five are central in this network and it is not possible to remove this ambiguity by calculating centrality in the aggregated network: in fact, all nodes in a clique have the same centrality and all have rank 1. Conversely, the multilayer analysis provides a unique versatile (most central) author, CC, solving the ambiguity raising with classical approaches. CC contributed only in two layers, at variance with the other authors who contributed in three layers, and therefore she is under-represented and consequently under-ranked when heuristics descriptors are employed. However, after a more careful inspection, CC is the only author bridging the two layers with the largest number of contributions and for this reason her role must be more central than other authors, even if they contributed in more layers. Full size image Versatility of nodes in empirical multilayer networks To show the results of our study, first we considered biologists, chemists, computer scientists, economists, inventors, mathematicians, philosophers and physicists in Wikipedia, and we built an interconnected multilayer network with 5,513 nodes where each layer represents a discipline and two people are connected if a hyperlink exists between their pages. The disciplines for each individual have been determined from the listed pages curated by the community on Wikipedia, whereas intra- and interlayer links are created as follows. First, we build the aggregated hyperlink network, regardless of the layer(s) each node belongs to: this network is directed and weighted by the number of hyperlinks between two web pages. We discard all nodes having total degree smaller than 4, regardless of the strength of the corresponding links, and we focus our attention only on nodes belonging to the giant connected component of the resulting network to build the multilayer. For example, if there exists a hyperlink between two scientists ( a and b ) and these happen to satisfy three disciplines simultaneously (physicists, philosophers and chemists), then we make three intralayer directed edges between a and b , one for each layer, uniformly distributing the weight of the hyperlink on each edge. If a and b do not share at least one layer, then directed interlayer edges are made between all pair of layers where a and b exist, with the weight of the original hyperlink uniformly distributed among such edges. Finally, interlayer edges between all nodes’ replicas are created and assigned weight 1. The ranking obtained from PageRank versatility is shown for some top nodes in Table 1 and is compared with the result of using the equivalent centrality measure in the aggregated version of the network. Note that Edward Osborne Wilson, the father of sociobiology, and Harold Clayton Urey, Nobel Prize in Chemistry, well known for theories on the development of organic life from non-living matter, who played a significant role in the development of the atom bomb,gained many positions with respect to the aggregated as well as, for instance, Kurt Gödel, one of the greatest logicians of all time, with impact on several different disciplines, from pure mathematics to physics and philosophy. Interestingly, our procedure captured the versatility of people generally recognized as trans -disciplinary, with outstanding contributions to different areas. This is the case of visionary people like Leonardo da Vinci (ranked 118 by PageRank), Italian genius who lived in the fifteenth century, and Leó Szilárd (480), who patented the idea of a nuclear reactor with Enrico Fermi and conceived fundamental tools in experimental research as the electron microscope, the linear accelerator and the cyclotron, who gained thousands of positions in the multilayer because of their relevance and their links to relevant people in multiple subjects. Versatility is successfully captured in Milton Friedman as well, contributing to economics, statistics, international finance, risk and insurance, and microeconomic theory, in Hilary Putnam, a computer scientist and mathematician with outstanding contributions in philosophy of mind, of mathematics and of science, and in Charles Stark Draper, an engineer and scientist who invented inertial navigation and founded the Massachusetts Institute of Technology’s Instrumentation Laboratory responsible for designing the guidance computer of NASA’s Apollo missions. In the aggregated network, the importance of bridging different subjects can not be accounted for and, as expected, very important, but not necessarily versatile, names are top ranked, Immanuel Kant (1), Aristotle (2), Plato (3), Thomas Aquinas (6), Isaac Newton (7) and Albert Einstein (9). We have performed similar analysis on the co-authorship network obtained from the papers published in journals of the American Physical Society between 2005 and 2009, from scientists working in European institutions (data provided by APS on request, https://publish.aps.org/datasets ). We considered also a sub-sample of two online social networks, Twitter and Instagram, and we built the multilayer network of 13,297 nodes, where two users are linked by directed and unweighted edges if they follow each other (see Supplementary Note 6 ). Table 1 PageRank Ranking. Full size table We also considered a transportation network (see ref. 26 for details about this data set and how it has been obtained) shown in Fig. 1b , 450 nodes and 37 layers, and found relevant differences between betweenness versatility and centrality in multilayer and aggregated networks, respectively. London airports are rather central in the aggregated network, although they become less important in the multilayer network, because they have many connections distributed on a few airlines. For the opposite reason, airports like Brussels and Paris Charles de Gaulle, less central in the aggregated, become versatile, because their flights are operated by almost all airlines (see Supplementary Tables 6–8 ). It is worth noting that, in general, there is not a linear relation between versatility and the number of layers where a node exists, because versatility also depends on the contribution of each node to its centrality per layer. For completeness, the rankings distributions are compiled in Supplementary Fig. 2 for all data sets. Centrality measures in this context play a crucial role in spreading processes, from epidemic transmission to delays’ propagation through airports [27] . We have explored the use of versatility to understand the role of nodes in substantial dynamical scenarios. Using the multilayer airport network above, we simulate ensembles of random walkers departing from each airport separately and calculate their coverage [15] at time τ , defined as the fraction of nodes that have been visited up to time τ . We use the coverage at time τ =1,000 as a proxy for the size of an hypothetical epidemic spreading [28] starting in an airport. In the absence of empirical data about the flow between different airports, it is difficult to assess the physical time scale of our simulations. We choose τ =1,000 as a good trade-off between the initial stage of the diffusion ( τ ≤100), where the dynamics is still very local and there is no difference between considering the multilayer network or its aggregation, and the final stage of the diffusion ( τ ≥10,000), where, conversely, the coverage is almost 100%, because diffusive agents had enough time to hit almost all airports in the network, with no difference between multilayer and aggregate networks. See Supplementary Note 7 for further details. We rank airports by their coverage and use PageRank versatility and PageRank centrality in the multilayer and aggregated networks, respectively, to predict it. The results are shown in Fig. 3a,b and put in evidence that PageRank versatility outperforms the predicting capabilities of the standard PageRank centrality obtained from the aggregated network. We have also considered another dynamical process that models airplane traffic on the airport network. The model is an extension of ref. 6 to multilayer networks. The traffic is simulated by injecting, at each time step, ρ airplanes at each airport with random destination. During the following time steps, airplanes travel to its destination using shortest routes over the multiplex structure. Each airport in each layer is attached with a queue where the airplanes wait to be routed. Airports will route airplanes considering its arrival time (first-in-first-out strategy). To simulate the physical constraints of the airports, each airport is assumed to have a limited routing capacity η (for the sake of simplicity we have considered the same value for all airports). Given a sufficiently large ρ , one or more airports will achieve a congested state. In that situation, the congested airports will not be able to handle the incoming traffic and the amount of airplanes waiting to be routed will increase proportional to time. Here, we analyse the ordering at which the airports arrive to congestion and we show how the betweenness versatility is a better predictor to this ordering than the betweenness centrality. See Supplementary Note 7 for further details. 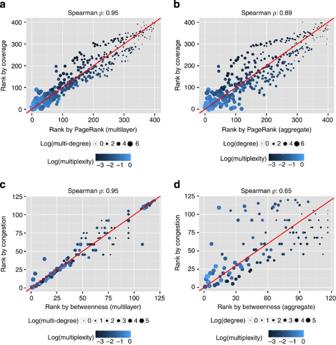Figure 3: Versatility as a predictor of nodes’ role in multilayer network dynamics. (a) We present the correlation between the coverage of random walkers15and the rank of the nodes by their Pagerank versatility using the multilayer structure. Inb, we present the correlation between the coverage of random walkers15and the rank of the nodes by their Pagerank centrality, using the aggregated structure. In all panels, we have used the multilayer airports network presented above (Fig. 1b), as a proxy of a plausible spreading. Points inaandbindicate the top 400 airports in terms of major coverage, their size is proportional to the degree and their colour encodes the fraction of airlines serving that airport (multiplexity). The red solid line is a guide for the eye of correlation equal to 100%. The aggregate descriptor is a good predictor (Spearman correlation is 89%) but it is not as significant as the versatility predictor (Spearman correlation is 95%). (c) We present the correlation between the congestion of simulated traffic of passengers with their betweenness versatility. (d) We present the correlation between the congestion of simulated traffic of passengers with their betweenness centrality. The top 120 airports are shown incandd. The aggregate descriptor (d) is not a good predictor (Spearman correlation is 65%) and it is outperformed significantly by the versatility predictor (Spearman correlation is 95%). Figure 3: Versatility as a predictor of nodes’ role in multilayer network dynamics. ( a ) We present the correlation between the coverage of random walkers [15] and the rank of the nodes by their Pagerank versatility using the multilayer structure. In b , we present the correlation between the coverage of random walkers [15] and the rank of the nodes by their Pagerank centrality, using the aggregated structure. In all panels, we have used the multilayer airports network presented above ( Fig. 1b ), as a proxy of a plausible spreading. Points in a and b indicate the top 400 airports in terms of major coverage, their size is proportional to the degree and their colour encodes the fraction of airlines serving that airport (multiplexity). The red solid line is a guide for the eye of correlation equal to 100%. The aggregate descriptor is a good predictor (Spearman correlation is 89%) but it is not as significant as the versatility predictor (Spearman correlation is 95%). ( c ) We present the correlation between the congestion of simulated traffic of passengers with their betweenness versatility. ( d ) We present the correlation between the congestion of simulated traffic of passengers with their betweenness centrality. The top 120 airports are shown in c and d . The aggregate descriptor ( d ) is not a good predictor (Spearman correlation is 65%) and it is outperformed significantly by the versatility predictor (Spearman correlation is 95%). Full size image We used betweenness versatility and betweenness centrality to predict the congestion ranking. We show the results in Fig. 3c,d , putting in evidence again that the versatility predictor outperforms the predictor obtained from the aggregated network. In summary, we have developed a framework to compute any centrality measure in the context of multilayer interconnected complex networks. These measures reveal the versatility of nodes according to a given definition. The versatility is proved to be a good descriptor of dynamical aspects on multilayer structures than can not be achieved considering the aggregation of layers into a single network. Versatility is a promising descriptor in the exploratory analysis of any categorized data set. How to cite this article : De Domenico, M. et al . Ranking in interconnected multilayer networks reveals versatile nodes. Nat. Commun. 6:6868 doi: 10.1038/ncomms7868 (2015).